Mild and selective hydrogenation of aromatic and aliphatic (di)nitriles with a well-defined iron pincer complex The catalytic hydrogenation of carboxylic acid derivatives represents an atom-efficient and clean reduction methodology in organic chemistry. More specifically, the selective hydrogenation of nitriles offers the possibility for a green synthesis of valuable primary amines. So far, this transformation lacks of useful, broadly applicable non-noble metal-based catalyst systems. In the present study, we describe a molecular-defined iron complex, which allows for the hydrogenation of aryl, alkyl, heterocyclic nitriles and dinitriles. By using an iron PNP pincer complex, we achieve very good functional group tolerance. Ester, ether, acetamido as well as amino substituents are not reduced in the presence of nitriles. Moreover, nitriles including an α,β-unsaturated double bond and halogenated derivatives are well tolerated in this reaction. Notably, our complex constitutes the first example of an homogeneous catalyst, which permits the selective hydrogenation of industrially important adipodinitrile to 1,6-hexamethylenediamine. The catalytic hydrogenation of carboxylic acid derivatives constitutes a major task for the development of green synthetic methodologies and is of actual importance in organic chemistry. Especially, in life science industries such transformations represent key technologies for the preparation of intermediates of new and existing pharmaceuticals as well as agrochemicals. So far, traditional reductions using (over)stoichiometric amounts of sensitive organometallic reagents prevail in this area. In particular, substituted nitriles lack of reliable reduction methods with molecular hydrogen, although they are easily accessible by a variety of reactions [1] , [2] , [3] , [4] , [5] , [6] , [7] . Furthermore, nitriles are readily available in nature: cyanogenic glycosides, cyan lipids and cyanohydrins are found in bacteria, algae, sponges and fungi as well as in higher organism [8] . In conventional organic synthesis, nitriles are typically reduced using stoichiometric amounts of metal hydrides [9] , [10] , hydrosilanes activated by a metal [11] , [12] , [13] or, more recently, organo-catalyst systems [14] . Clearly, all these methods suffer from poor atom efficiency and large waste production. Furthermore, owing to their high reactivity metal hydrides reveal only limited functional group selectivity. Although hydrosilylations show improved tolerance for a variety of substituents, expensive hydrosilanes are required in equimolar amounts. Undoubtedly, the selective hydrogenation represents a more economic and sustainable route to valuable primary amines. On the one hand, heterogeneous materials are well studied and commonly used for nitrile hydrogenation in industry. In these cases, mainly catalysts based on Co and Ni are utilized, which usually provide good selectivities for ‘simple’ substrates [15] , [16] , [17] . In addition, in academia a variety of transition metals including Co, Ni, Au [18] , Cu, Rh, Pd and Pt have been immobilized on different supports (C, TiO 2 , SiO 4 , Al 2 O 3 and so on) and were investigated, too [19] , [20] , [21] , [22] , [23] , [25] . On the other hand, homogeneous catalysts for the hydrogenation of nitriles are almost limited to the presence of precious metals such as Ir [26] , Rh [27] , Re [28] and Ru [29] , [30] , [31] , [32] , [33] , [34] . First detailed studies on the hydrogenation of nitriles in the presence homogeneous catalysts were performed by Pez [35] and Grey [36] in the early 80’s. Recent progress is mainly achieved using ruthenium-based catalysts, which is also highlighted in a patent by Beatty and Paciello [37] . Particularly, different Ru complexes were reported by Morris et al . [29] , Sabo-Etienne and co-worker [33] , Leitner’s group [30] , Bruneau et al . [31] and our group in the last decade [34] , [38] , [39] . Most of these catalytic systems make use of P - or PN -ligands requiring the addition of base to prevent side reactions. It should be noted that until now only one non-precious metal catalyst based on Ni has been reported for the reduction of nitriles. Unfortunately, the desired amine was obtained only as a side product [40] . Hence, there is still a strong need to develop new and improved catalyst systems for this transformation. In addition to specific polymers, the vast majority of today’s pharmaceuticals and agrochemicals contain amino groups [41] . In Fig. 1 , the bulk polymer Nylon-6,6 and a small selection of pharmaceuticals are shown. Thus, the synthesis of primary amines and particularly primary diamines are of significant interest as intermediates in academic and industrial research [15] , [42] , [43] , [44] , [45] . These products can easily be modified by follow-up reactions to obtain secondary amines, for example, via reductive amination or N -methylation, representing useful active drugs. Although several novel catalytic methods for the synthesis of primary amines have been established in the past decades [13] , [46] , [47] , [48] , [49] , [50] , [51] , [52] , their preparation remains challenging due to the higher reactivity compared with the secondary and tertiary derivatives. 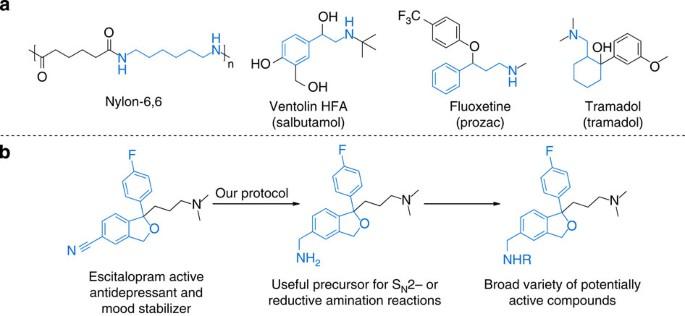Figure 1: Amino-containing pharmaceuticals. (a) Selection of important amino-containing pharmaceuticals and polymers; (b) hydrogenation of Escitalopram. Figure 1: Amino-containing pharmaceuticals. ( a ) Selection of important amino-containing pharmaceuticals and polymers; ( b ) hydrogenation of Escitalopram. Full size image Herein, we describe the first selective iron-catalysed hydrogenation of nitriles. Advantageously, in our straightforward, atom efficient and environmentally friendly protocol, no additives are needed. Besides the common (hetero)aromatic and aliphatic nitriles, we were able to hydrogenate successfully also dinitriles such as the industrially important adipodinitrile. Influence of important reaction parameters On the basis of previous efforts on the reduction of carboxylic acid derivatives [6] , [53] , [54] , [56] and our continuing interest in the development of non-precious metal catalysts [57] , [58] , [59] , [60] , [61] , [62] , [63] , [64] , [65] , [66] , we started a programme to study base metal-catalysed reductions of nitriles. Among the different catalysts tested, the well-defined iron pincer complex 3 (refs 59 , 67 ) revealed some activity. Recently, another access to this complex was reported by Schneider et al . [68] and a related Co-based Pincer type catalyst has been described for reductions of imines, carbonyl compounds and olefins [69] . Therefore, we investigated this PNP pincer complex in more detail. For our initial studies, we used the benchmark reaction of 4-phenylbenzonitrile to obtain 4-phenylbenzyl amine. To evaluate the factors responsible for the formation of primary amines, we examined the influence of different solvents, temperatures and catalyst loadings. Selected experiments are shown in Table 1 . All hydrogenation reactions were performed in an eightfold parallel autoclave charged with 4-ml glass vials. Interestingly, we observed a strong influence of the solvent. Excellent conversion but no desired selectivity was obtained using THF as solvent. Here, several by-products such as imine, bis-imine, bis-amine and even an aldehyde were formed at elevated temperatures of 100 °C ( Table 1 , entries 2 and 3). As an exception, benzonitrile as well as 4-methoxybenzonitrile could be hydrogenated in THF with high yields of 93 and 97%, respectively. Applying dichloromethane, aromatic solvents or DMF, no reactivity was observed. Gratifyingly, using alcohols as solvents gave both high reactivity and selectivity for the primary amine ( Table 1 , entries 9 and 10). The high hydrogenation activity of the iron catalyst is demonstrated by full conversion and excellent selectivity applying only 70 °C reaction temperature ( Table 1 , entry 13). However, at 40 °C the catalytic activity dropped and lower conversion was obtained ( Table 1 , entry 14). Notably, for successful reduction hydrogen is required, while transfer hydrogenation can be excluded ( Table 1 , entry 12). Table 1 Catalytic hydrogenation of 4-phenylbenzonitrile: variation of solvents and temperatures*. Full size table Substrate scope for (hetero)aromatic nitriles With optimized reaction parameters in hand ( i PrOH, 70 °C, 30 bar H 2 and 3 h), we were interested in the generality of this iron-catalysed hydrogenation of nitriles. Therefore, we examined various (hetero)aromatic substrates. 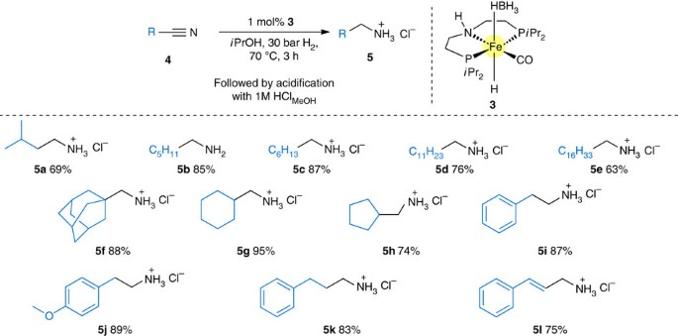Figure 2: Fe-catalysed hydrogenation of aliphatic nitriles. Reaction Conditions:0.5 mmol nitrile, 0.005 mmol3, 1 mliPrOH, 30 bar H2, 70 °C, 3 h; conversion (>99%) determined by GC. Yield was determined as isolated HCl salt. Yield of5bwas determined by GC using hexadecane as internal standard. As shown in Table 2 , arenes with electron-donating substituents were hydrogenated with good to excellent isolated yields (up to 99%) ( Table 2 , entries 1–10). Catalytic hydrogenation of benzonitriles containing electron-withdrawing groups like halogens, esters and heteroaromatic nitriles progressed well at 100 °C. Hence, different substituted CF 3 -, fluoro- and bromo-benzonitriles furnished yields from 71 to 92% ( Table 2 , entries 12, 13, 15 and 16). In addition, sulphur- and nitrogen-containing heteroaromatic nitriles ( Table 2 , entries 17–20) were isolated in yields up to 92%. Among the electron-deficient nitriles, 4-chlorobenzonitrile, methyl 6-methoxynicotinonitrile and 4-cyanobenzoate provided some Schiff base side products at 100 °C ( Table 2 , entries 14, 18 and 21). However, at higher temperature of 130 °C, the formation of the Schiff base was prevented to give selectively the primary amine. Table 2 Catalytic hydrogenation of various aromatic nitriles: scope and limitation*. Full size table Exploring our catalytic protocol with more substrates containing functional groups like ester, nitro, amine, hydroxy, acetamide and cyanide, we obtained very good results for ester, acetamide and amine substituents on the aromatic ring ( Table 2 , entries 21–23). Nevertheless, nitro- and hydroxy-containing benzonitriles did not show any conversion under the present conditions. We assume that the hydrogenation of 4-hydroxybenzonitrile is probably hindered due to interactions of the free hydroxyl-group with the catalyst. Substrate scope for aliphatic nitriles Furthermore, the reaction was carried out in the presence of the more challenging aliphatic nitriles, furnishing 12 desired primary amines in good to excellent isolated yields up to 95% running the reaction at 70 °C ( Fig. 2 ). At this point, it is important to note that catalytic hydrogenations of aliphatic nitriles are much less investigated due to base-induced side reactions using common hydrogenation catalysts. In addition, cyclic aliphatic nitriles were easily reduced in good to very good yields. For the interesting substrate cinnamonitrile 4l , we found very good selectivity for the nitrile hydrogenation without reducing the C-C double bond (>25:1). This result illustrates that it is possible to reduce a nitrile moiety in the presence of an α,β-unsaturated double bond using our catalyst system furnishing synthetically important allylic amines. Figure 2: Fe-catalysed hydrogenation of aliphatic nitriles. Reaction Conditions: 0.5 mmol nitrile, 0.005 mmol 3 , 1 ml i PrOH, 30 bar H 2 , 70 °C, 3 h; conversion (>99%) determined by GC. Yield was determined as isolated HCl salt. Yield of 5b was determined by GC using hexadecane as internal standard. Full size image Hydrogenation of dinitriles Finally, the hydrogenation of industrially relevant dinitriles was explored. As an example, adipodinitrile was investigated that is annually hydrogenated at elevated pressures in the polymer industry on mio-ton scale to give 1,6-hexamethylenediamine (1,6-HMD) as an essential building block for the production of Nylon-6,6 (refs 45 , 70 ) In this case, it is essential to achieve the diamine in high purity to prevent side-reactions during the polymerization process [25] . 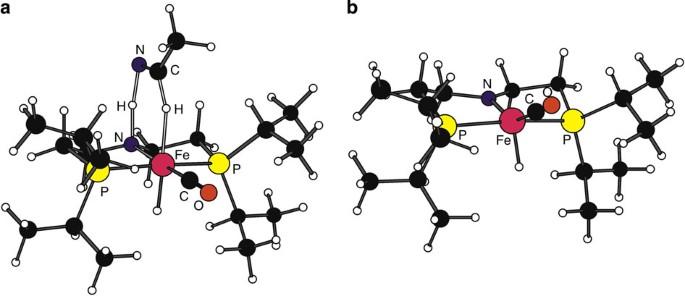Figure 3: Catalytic intermediates. (a) transition state of the protic hydrogen to the nitrile-nitrogen and hydride coordination to the corresponding carbon; (b) dehydrogenated complex9. Using our standard protocol, we obtained the desired 1,6-hexamethyldiamine in excellent yields (95%) and high NMR purity ( Table 3 , entry 1). Up-scaling of the reaction by factor of 50 in the presence of low catalyst loading (0.5 mol%) also provided 1,6-HMD in similar isolated yield and a TON of 174 ( Table 3 , entry 2). Noteworthy, the reduction of adipodinitrile attained nearly full conversion after only 20 min giving 83% yield of the isolated HCl salt product with a TON of 83 and a TOF of 250 h −1 ( Table 3 , entry 3). Table 3 Catalytic hydrogenation of dinitriles 6*. Full size table Similar to adipodinitrile, the hydrogenation of terephthalodinitrile gave the corresponding diamine in high isolated yield of 85% ( Table 3 , entry 5, 7c ). This finding matches well with the observed yields for other electron-deficient aromatic nitriles shown in Table 3 . Furthermore, a branched aliphatic dinitrile was reduced to the respective diamine, albeit with a lower selectivity due to the formation of side products as the bis-imine and the mono-reduction product ( Table 3 , entry 4, 7b ). DFT calculations Next, we became interested in elucidating the possible reaction mechanism for this nitrile reduction. We have carried out B3PW91 density functional theory computation along with the TZVP all-electron basis set as well as spectroscopic studies vide supra . In our computations, we explored the inner-sphere and outer-sphere hydrogenation mechanisms by using the real size complex 8 (complex 3 without BH 3 ) as well as acetonitrile and benzonitrile as model substrates. All computational details are given in the Supporting Information (see Supplementary Method 1 and Supplementary Data 1 ), and only the essential results are discussed and compared here. In the inner-sphere mechanism, the first step is CO dissociation to create a free site for nitrile coordination and subsequent hydrogenation. In the outer-sphere mechanism, a free coordination site is not necessary, and the nitrile is hydrogenated directly to the imine, which is further reduced to the amine. More specifically, our computations show that CO dissociation from complex 8 is highly endergonic by 23.78 kcal mol −1 . However, it is interesting to note that the coordination of acetone and benzonitrile to the complex (a triplet ground state) after CO dissociation is endergonic by 9.91 and 7.19 kcal mol −1 , respectively. This reveals that nitriles cannot replace the CO ligand and therefore dissociation is not preferred. In the outer-sphere mechanism, the computed activation free energy for the concerted nitrile hydrogenation to imine is 17.55 and 15.35 kcal mol −1 for acetonitrile and benzonitrile, respectively. These barriers are lower than the CO dissociation energy by 6.23 and 8.43 kcal mol −1 , respectively. Figure 3a shows the transition state for acetonitrile coordination in the outer-sphere mechanism. Figure 3: Catalytic intermediates. ( a ) transition state of the protic hydrogen to the nitrile-nitrogen and hydride coordination to the corresponding carbon; ( b ) dehydrogenated complex 9 . Full size image In addition, the hydrogenation of acetonitrile and benzonitrile to the corresponding imine is exergonic by 0.96 and 4.10 kcal mol −1 , respectively. This energetic difference demonstrates the preference of the outer-sphere mechanism over the inner-sphere mechanism. The hydrogenation of the nitrile to give the desired amine proceeds in two reduction steps. In the first cycle an imine is formed, which subsequently gives the corresponding amine. In both reactions, the important catalytic intermediate is the dehydrogenated complex ( 9 , Fig. 3 ), which represents a singlet ground state (more stable than the triplet state by 13.90 kcal mol −1 ). Natural bond orbital analysis reveals a Fe-N single bond in 8 and a Fe=N double bond in 9 with the respective Fe-N bond orders 0.350 for 8 and 0.688 for 9 . It is found that the regeneration of complex 8 from intermediate 9 has an activation free energy barrier of 17.14 kcal mol −1 , and the reaction is slightly exergonic by 0.33 kcal mol −1 . This indicates the facile reversibility of the dehydrogenation and hydrogenation of complex 8 . In contrast to the first step from nitrile to imine, the second step from imine to amine is indeed without barrier. Attempts to find this barrier resulted only in the direct formation of free amine, which is exergonic by 14.04 and 11.18 kcal mol −1 for ethanimine and phenylmethanimine (see the reaction profile in SI, Supplementary Fig. 1 ), respectively. Infrared measurements To confirm that CO remains on the iron centre during the catalysis, we performed infrared measurements for the hydrogenation of benzonitrile to benzyl amine (conditions: 10 mol% 3 , 100 °C, 3 h, 30 bar H 2 , Supplementary Method 2 ). After the reaction was completed (> 99% conversion), we evaporated the solvent very slowly and recorded the appropriate infrared spectra (see SI, Supplementary Fig. 2 ). Indeed, the CO band of a ligated iron carbonyl complex appears with a wavenumber of ν =1,898 cm −1 . Without any solvent present, complex 3 shows the CO band at ν =1,891 cm −1 . This finding confirmed the assumption that the ligated iron carbonyl complexes still exist after the reaction. Control experiments Furthermore, to support the statement that an outer-sphere mechanism takes place and to demonstrate the critical role played by the N-H group of the PNHP i Pr ligand, we synthesized the iron(II) complex analogue of 3 , Me-3 (for NMR spectra see Supplementary Fig. 3a–f , for NMR analysis see Supplementary Methods 3 ), containing the ligand PNMeP i Pr (PNMeP i Pr=bis[(2-diisopropylphosphino)ethyl]methyl amine). Here, the hydrogen of the nitrogen in the ligand is replaced by a methyl group. As shown in Fig. 4a , no conversion was observed when this iron complex Me-3 was applied in the hydrogenation of 4-phenylbenzonitrile. 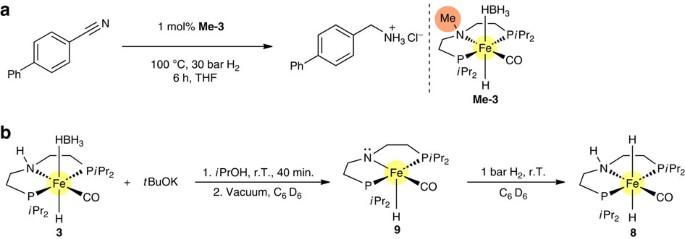Figure 4: Mechanistic studies. (a) Hydrogenation of 4-phenylbenzontrile withMe-3; (b) synthesis of amido complex9and dihydride8. Figure 4: Mechanistic studies. ( a ) Hydrogenation of 4-phenylbenzontrile with Me-3 ; ( b ) synthesis of amido complex 9 and dihydride 8 . Full size image NMR investigations In agreement with the calculations, the dihydride species 8 and amido complex 9 were observed by NMR when a solution of the catalyst precursor 3 and benzonitrile 1a in THF- d 8 was heated to 60 °C under a hydrogen atmosphere. Their identity was confidently assessed by comparison with samples of 8 and 9 prepared via an alternative route from 3 according to Fig. 4b (see SI for NMR spectra, Supplementary Figs 4–11 ). The amido complex 9 is extremely oxygen sensitive and was not isolated. However, these compounds cannot be isolated because, on solvent removal under reduced pressure, it turns back into the amido complex. On exposure of the NMR sample to hydrogen (1 bar), the dihydride complex 8 is formed which, however, is only stable under hydrogen atmosphere and reverts back to the amido complex 9 by loss of H 2 . This equilibrium can also be shifted by heating to the amido complex 9 . 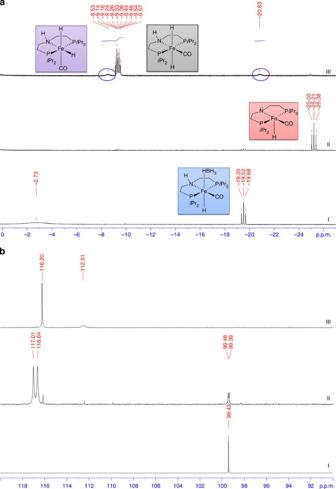Figure 5: NMR studies. (a)1H NMR spectra (benzene-d6, hydride region) of catalyst precursor3(I, 300.1 MHz), amido complex9(II, 300.1 MHz) and dihydride8(III, 400.1 MHz); (b)31P{1H }NMR spectra (benzene-d6) of catalyst precursor3(I, 121.0 MHz), amido complex9(II, 121.0 MHz, residual coupling to hydride hydrogens is present) and dihydride8(III, 161.9 MHz). Figure 5 shows the 1 H NMR (hydride region) and 31 P{ 1 H} NMR spectra of species 8 (spectra III) and 9 (spectra III) as compared with the catalyst precursor 3 (spectra I), respectively. Besides the trans -dihydride complex 8 , spectra II also shows the presence of a second species. On cooling the sample, the broad signals turned into two well-defined triplets of doublets that couple to each other, J HH =15.4 Hz, and to the two phosphorus of the ligand, most probably accounting for the cis - 8 dihydride, having the two hydrides cis relative to each other (see also Supplementary Figs 12–17 ). Figure 5: NMR studies. ( a ) 1 H NMR spectra (benzene- d 6 , hydride region) of catalyst precursor 3 (I, 300.1 MHz), amido complex 9 (II, 300.1 MHz) and dihydride 8 (III, 400.1 MHz); ( b ) 31 P{ 1 H }NMR spectra (benzene- d 6 ) of catalyst precursor 3 (I, 121.0 MHz), amido complex 9 (II, 121.0 MHz, residual coupling to hydride hydrogens is present) and dihydride 8 (III, 161.9 MHz). Full size image The corresponding data are presented in Table 4 . These data compare favourably with those of the analogous Fe species reported by Milstein [69] containing the pyridine-based ligand 2,6-bis((diisopropylphosphanyl)-methyl)pyridine. Table 4 1 H (hydride region) and 31 P NMR data of complexes 3 , 8 and 9 in benzene- d 6. . Full size table In light of the obtained results, we suggest the following mechanism ( Fig. 6 ). As a first step of catalyst activation, we assume the loss of BH 3 to give complex 8 . Then, the nitrile is hydrogenated in a concerted way by a simultaneous transfer of the hydride from the iron centre and the proton from the nitrogen ligand to give the corresponding imine 10 and the amido complex 9 . The dihydrido species 8 is regenerated by the addition of molecular hydrogen. The imine 10 undergoes a second reaction cycle and is finally reduced to the corresponding amine 2 . 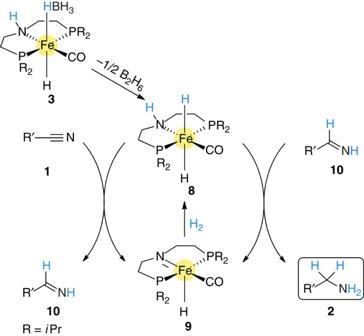Figure 6: Proposed mechanism. Proposed mechanism for nitrile reduction with complex8(=complex3without BH3). Figure 6: Proposed mechanism. Proposed mechanism for nitrile reduction with complex 8 (=complex 3 without BH 3 ). Full size image In summary, we have developed the first iron-catalysed hydrogenation of aliphatic and (hetero)aromatic (di)nitriles to yield the corresponding primary amines in good to excellent yields. This methodology proceeds with high chemoselectivity even in the presence of other reducible functional groups like ester, amido and α,β-unsaturated double bonds. In contrast to most known catalytic hydrogenations of nitriles, the iron complex 3 is active without additional base. This is an important advantage compared with known homogeneous catalyst systems. Another important aspect of the present work is the selective reduction of dinitriles using molecular hydrogen. As a highlight, the efficient hydrogenation of adipodinitrile towards 1,6-HMD proceeds under mild conditions in a short time. On the basis of calculations and spectroscopic investigations, we propose an outer-sphere mechanism for a concerted nitrile hydrogenation. Finally, it is worth noting that the pincer-type PNP iron catalyst represents the first non-precious catalyst for a general hydrogenation of nitriles. The broad applicability and the relatively mild reaction conditions make this procedure interesting for the synthesis of all kinds of fine and bulk chemicals. General analytic methods Unless otherwise stated, all reaction mixtures were prepared in 4-ml glass vials under an argon atmosphere with exclusion of moisture from reagents and glassware using standard techniques for manipulating air-sensitive compounds. Reactions were carried out in eightfold 300-ml autoclaves (PARR Instrument) under a hydrogen atmosphere. All isolated compounds were characterized by 1 H NMR and 13 C NMR spectroscopy, GCMS and HRMS. NMR spectra were recorded on Bruker AV 300/400. In 31 P NMR spectra, chemical shifts ( δ ) are reported in p.p.m. relative to 85% H 3 PO 4 as external standard. All chemical shifts ( δ ) are reported in p.p.m. and coupling constants ( J ) in Hz. All chemical shifts are related to solvent peaks (DMSO- d 6 : 2.5 ( 1 H), 39.52 ( 13 C), D 2 O- d 2 : 4.80 ( 1 H) or methanol- d 4 : 3.3 ( 1 H), 49.0 ( 13 C), THF- d 8 : 3.58 ( 1 H), benzene- d 6 : 7.16 ( 1 H), 128.06 ( 13 C)), respectively. All measurements were carried out at room temperature unless otherwise stated. Mass spectra were in general recorded on a Finnigan MAT 95-XP (Thermo Electron) or on a 6210 Time-of-Flight LC/MS (Agilent). Gas chromatography was performed on a HP 6890 with a HP5 column (Agilent). Infrared spectra were recorded on Alpha spectrometer (Bruker) using the ATR method. The wavenumbers are reported in cm −1 . Reagents Unless otherwise stated, commercial reagents were used without purification. Hydrogenation of Nitriles Under an argon atmosphere a 4-ml glass vial equipped with a cap, septum, needle and stirring bar was charged with 3 (0.005 mmol) and diluted in 1 ml iso -propanol (degassed). After a short stirring, the nitrile (0.5 mmol) was added under argon. The vial was placed into the alloy plate in the autoclave. The apparatus was purged three times with hydrogen, pressurized to 30 bar H 2 , and stirred for 3 h at 70, 100 or 130 °C. Afterwards, the autoclave was cooled to room temperature, depressurized and the reaction mixture was analysed by GC and isolated HCl salt by NMR, GC–MS and HRMS. For NMR and GC–MS/HR-MS analysis see Supplementary Method 4 . Isolation as HCl salt: the reaction mixture was diluted in a large amount (~50 ml) of diethyl ether before 1 ml of 1 M HCl MeOH solution was added. A precipitation occurred immediately, which was filtered and washed with diethyl ether and ethyl acetate. For 1 H and 13 C NMR spectra of selected compounds, see Supplementary Figs 18–30 . Synthesis of Me-3 and intermediates Synthesis of (CH 3 )N((CH 2 CH 2 )P(CH(CH 3 ) 2 ) 2 ) 2 In a flame dried and argon flushed 100-ml Schlenk flask, 10 g of a 10% w/w solution of di-isopropyl phosphine (8.46 mmol, 2.0 equiv.) was dissolved in 10 ml diethyl ether. After cooling to −78 °C, 5.3 ml of a 1.6 M in hexane butyl lithium solution (8.46 mmol, 2.0 equiv.) was added dropwise under constant stirring. The reaction mixture was allowed to reach room temperature, and the Schlenk flask was equipped with a reflux condenser and heated for 4 h at reflux under an argon atmosphere, during which time a white solid was formed. In a flame dried and argon flushed 50-ml Schlenk flask, 0.815 g (4.23 mmol, 1.0 equiv.) N -methyl bis(2-chloroethyl)amine hydrochloride was dissolved in 10 ml diethyl ether and cooled to −78 °C. Under constant stirring, 2.9 ml of a 1.6 M in hexane butyl lithium solution was added dropwise. After allowing the reaction mixture to reach room temperature, the content was stirred for 2 h and then transferred slowly via a transfer cannula to the precooled di-isopropyl phosphine lithium suspension in the 100-ml Schlenk flask at −78 °C. The resulting reaction mixture was allowed to reach room temperature and then refluxed overnight under an argon atmosphere. The reaction mixture was cooled down to room temperature and 20 ml of degassed water was added. The aqueous layer was decanted by cannula and the organic layer was further washed with two portions of degassed water (2 × 15 ml). The organic phase was then dried over sodium sulphate. After stirring for 1 h, the sodium sulphate was filtered off through a short plug of silica gel and the solvent removed in vacuum to yield a colourless liquid (0.860 mg, 2.69 mmol, 96% purity according to 31 P NMR, 61% yield). The ligand was used without further purification. Synthesis of {Fe(H)(HBH 3 )[(CH 3 )N((CH 2 CH 2 )P(CH(CH 3 ) 2 ) 2 ) 2 ]} A solution of (CH 3 )N((CH 2 CH 2 )P(CH(CH 3 ) 2 ) 2 ) 2 (2.15 mg, 0.67 mmol, 1 equiv.) in 1 ml n -heptane was added dropwise to a solution of anhydrous FeBr 2 (145 mg, 0.67 mmol, 1 equiv.) in 40 ml THF. The resulting solution was stirred at room temperature for 4 h. The solution was concentrated and n -heptane added. The resulting mixture was stirred vigorously until an off-white precipitate was formed. The solvent was decanted and the solid washed with two further portions of n -heptane. It was then dried under vacuum and used as such for the next step. {FeBr 2 [(CH 3 )N((CH 2 CH 2 )P(CH(CH 3 ) 2 ) 2 ) 2 ]} was dissolved in a mixture of MeCN (5 ml) and EtOH (15 ml) to give a clear deep purple solution. The solution was cooled to 0 °C and NaBH 4 (102 mg, 2.69 mmol, 4 equiv.) was added in one portion. Gas evolution took place and the solution turned dark brown. It was then stirred at room temperature for 3 h. After this time, the solvent was removed in vacuum. The residue was extracted with n -heptane, and the resulting mixture filtered through a short plug of celite to give a clear dark brown solution. The solvent was removed in vacuum to give a dark brown solid, which was dried under high vacuum overnight, 170 mg (0.43 mmol, 64% yield). Synthesis of {Fe(H)(HBH 3 )(CO)[(CH 3 )N((CH 2 CH 2 )P(CH(CH 3 ) 2 ) 2 ) 2 ]} {Fe(H)(HBH 3 )[(CH 3 )N((CH 2 CH 2 )P(CH(CH 3 ) 2 ) 2 ) 2 ]} (170 mg, 0.43 mmol) was dissolved in 30 ml THF to give a clear dark brown solution. CO was bubbled through until the solution turned bright yellow. Solvent was removed under vacuum to provide a yellow residue. NMR analysis of the crude product showed the presence of {Fe(H) 2 (CO)[(CH 3 )N((CH 2 CH 2 )P(CH(CH 3 ) 2 ) 2 ) 2 ]} and {Fe(H)(HBH 3 )(CO)[(CH 3 )N((CH 2 CH 2 )P(CH(CH 3 ) 2 ) 2 ) 2 ]}. The residue was extracted with n -heptane, and the resulting suspension was filtered through a short plug of celite. Solvent was removed under vacuum to leave a yellow solid of {Fe(H) 2 (CO)[(CH 3 )N((CH 2 CH 2 )P(CH(CH 3 ) 2 ) 2 ) 2 ]} (35 mg, 0.086 mmol); the residue left after n -heptane extraction was dissolved in toluene and filtered as well through celite. Removal of the solvent under vacuum afforded 86 mg, 0.205 mmol, of {Fe(H)(HBH 3 )(CO)[(CH 3 )N((CH 2 CH 2 )P(CH(CH 3 ) 2 ) 2 ) 2 ]}, which, however, contained 12% of {Fe(H) 2 (CO)[(CH 3 )N((CH 2 CH 2 )P(CH(CH 3 ) 2 ) 2 ) 2 ]} according to 31 P NMR (overall yield 68%). How to cite this article: Bornschein, C. et al . Mild and selective hydrogenation of aromatic and aliphatic (di)nitriles with a well-defined iron pincer complex. Nat. Commun. 5:4111 doi: 10.1038/ncomms5111 (2014).